Arrays ofLuciusmicroprisms for directional allocation of light and autostereoscopic three-dimensional displays Directional and asymmetric properties are attractive features in nature that have proven useful for directional wetting, directional flow of liquids and artificial dry adhesion. Here we demonstrate that an optically asymmetric structure can be exploited to guide light with directionality. The Lucius prism array presented here has two distinct properties: the directional transmission of light and the disproportionation of light intensity. These allow the illumination of objects only in desired directions. Set up as an array, the Lucius prism can function as an autostereoscopic three-dimensional display. Many biological systems show intriguing directional and asymmetric structures for specific functions [1] , [2] , [3] , [4] , [5] , [6] , [7] , [8] , [9] . Examples include the directional water collection on periodic spindle knots in spider silk [1] and the adhesion hysteresis of hierarchically organized slanted hairs on gecko's feet [6] , [7] , [8] , [9] . These structures provide unique functions, such as the difference in contact angles on the asymmetric structure and the change in adhesion force depending on pulling direction with the help of the structural modulation of surface and interfacial properties. Here, we use an array of microscale prisms with optical asymmetry to guide light directionally. The operating principles are based on the basic geometrical optics of transmission, reflection and refraction of incident light rays [10] . The prism array has one or more prism faces made reflective or black by coating with a suitable material, such as metal, whereas the other faces remain transparent. For a typical triangular prism, one face is reflective or absorbent, and the other two faces are transparent. With recent advances in microfabrication technologies, a triangular prism having a reflective or black film on one side can be easily fabricated in a miniaturized shape. Using such a prism array—which we term a Lucius prism—we can see an object only in the desired direction. Thus, by simply placing a Lucius prism on a screen, it can be made to permit only frontal viewing. The disproportionation of light intensity allows the allocation of light in any desired direction, such that two distinctly different images can be shown to the left and right eyes without the need of special viewing eyewear, an essential feature of autostereoscopic three-dimensional (3D) displays. 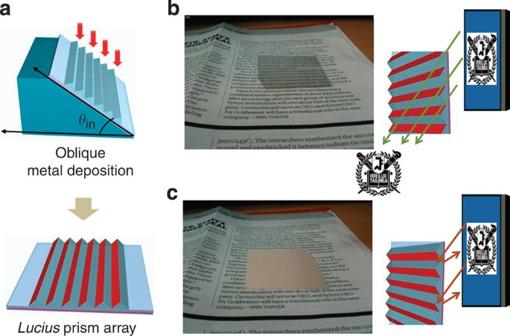Figure 1: Directional transmission of light by aLuciusprism array. (a) A schematic illustration of fabrication concept for preparing aLuciusprism array sheet. (b) When the prism sheet is placed on a newspaper in the right direction, the letters in the newspaper are visible because the light travels in the direction parallel to the reflective metal film. (c) When we rotate the prism sheet, it becomes reflective because the travelling light is reflected off the deposited metal film. Fabrication of the Lucius prism array The fabrication of the Lucius prism array is illustrated in Figure 1a . First, a prism film sheet is prepared with the aid of replica moulding. For this purpose, a master or template was prepared by the diamond-tool machining of an electroplated nickel plate into an array of microprisms. Drops of a prepolymer solution of polyurethane acrylate (PUA) were dispensed onto this template, and the film was lightly pressed with a polyethylene terephthalate (PET) backplane sheet. Exposure to ultraviolet light cures the prepolymer [11] . The PET sheet removed from the template has an array of PUA prisms on its surface. This polymer prism sheet was then coated with metal of 100–300 nm thickness on only one side of the prisms using oblique metal deposition. For the deposition, the transparent prism sheet was placed on an inclined holder ( θ in in Fig. 1a , henceforth to be referred to as the oblique angle) in a thermal or electron gun evaporator maintained at 10 −6 Torr. The oblique deposition, which has been widely used to create smart micro- or nanostructures in various applications [2] , [3] , [12] , [13] , [14] , [15] , [16] , [17] , completes the fabrication of the Lucius prism array ( Supplementary Fig. S1 ). Figure 1: Directional transmission of light by a Lucius prism array. ( a ) A schematic illustration of fabrication concept for preparing a Lucius prism array sheet. ( b ) When the prism sheet is placed on a newspaper in the right direction, the letters in the newspaper are visible because the light travels in the direction parallel to the reflective metal film. ( c ) When we rotate the prism sheet, it becomes reflective because the travelling light is reflected off the deposited metal film. Full size image Directional transmission of light by the Lucius prism array The directional transmission of light made possible by the Lucius prism array can best be demonstrated by placing the prism sheet on a newspaper. Here, a reflective metal layer of aluminium (Al; 100–200 nm thickness) was obliquely deposited on one side of the prism array. When the prism sheet is placed in such a way that the transmitted light is parallel to the reflective metal-deposited face, the letters on the newspaper are clearly visible because the sheet is transparent in that direction ( Fig. 1b ). When the sheet is rotated by 180°, however, the film becomes reflective, and the letters are no longer visible ( Fig. 1c ). This change from a transparent film to a mirror is due to the structural characteristics of the Lucius prism array, as schematically illustrated on the right-hand sides of Figure 1b,c . As the prism sheet is rotated, the corresponding transmission level is modulated ( Supplementary Movie 1 ). A Lucius prism array allowing only frontal viewing The directional transmission capability of a Lucius prism array can also be exploited for frontal viewing using the same prism structure shown in Figure 1 . 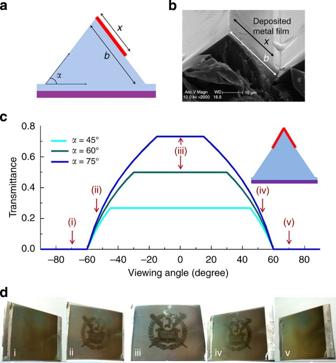Figure 2:Luciusprism array allowing only frontal viewing. (a) A single prism partially covered with a metal film on one side. (b) A SEM image of a prism array when the incidence angle of the metal deposition is 50°. The picture shows that the metal film does not cover the whole prism surface. (c) Transmittance of incident light as a function of the viewing angle (θview). The plots were based on equations (1–3) assuming that metal films partially cover both sides of the prism in symmetric fashion, as schematically shown on the right side of the figure. (d) Pictures of the SNU logo as seen at different viewing angles numbered (i) through (v) inFigure 2cwhen theLuciusprism sheet was placed on top of the logo. If we use the notation given in Figure 2a , the coverage, x / b , which is defined as the fraction of a surface of one side of the prism deposited with a metal film as measured from the prism apex down, is determined solely by the oblique angle θ in and the prism angle α (refer to Fig. 2a ). The relationship of the coverage is derived in Supplementary Figure S2 . A scanning electron microscopy (SEM) image of a partially covered prism surface is shown in Figure 2b , in which the geometric configuration with θ in =50° and α =45° was employed. If anything is to be visible through the prism sheet, the prisms must be partially covered with a metal film because, otherwise, the whole surface becomes reflective, and nothing is visible. For frontal viewing, a symmetry must exist with respect to the surface coverage simply because the image beneath the Lucius prism sheet should not be seen from either the left or the right side. Such a symmetric prism surface coverage, as schematically illustrated in Figure 2c , can be obtained by repeating the oblique deposition twice, once on one side and then repeated on the other side of the prism array. A SEM image of the symmetric prism structure is given in Supplementary Figure S3 . Figure 2: Lucius prism array allowing only frontal viewing. ( a ) A single prism partially covered with a metal film on one side. ( b ) A SEM image of a prism array when the incidence angle of the metal deposition is 50°. The picture shows that the metal film does not cover the whole prism surface. ( c ) Transmittance of incident light as a function of the viewing angle ( θ view ). The plots were based on equations (1–3) assuming that metal films partially cover both sides of the prism in symmetric fashion, as schematically shown on the right side of the figure. ( d ) Pictures of the SNU logo as seen at different viewing angles numbered (i) through (v) in Figure 2c when the Lucius prism sheet was placed on top of the logo. Full size image It can be shown (in Supplementary Fig. S4a ) that the transmittance T is zero if the viewing angle ( θ view ) is larger than the oblique angle θ in , that is, Here, the viewing angle θ view is defined such that it is zero for the frontal view, negative in the counterclockwise direction and positive in the clockwise direction. The transmittance for the viewing angle less than θ in can be derived, as detailed in Supplementary Figure S4b and S4c , to yield The above equations show that the transmittance is constant at the value given by equation (2) for a viewing angle less than 90− α , including zero or frontal viewing angles, and then decreases to zero towards the viewing angle close to the oblique angle, as shown in equation (3). 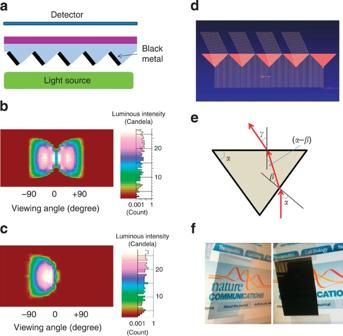Figure 3: Disproportionation of intensity of incident light. (a) A schematic illustration of aLuciusprism sheet placed between a light source and a detector for the disproportionation of incident light intensity. (b) Isoluminance contour plot obtained by a simulation tool. Note that the intensity distribution through the normal prism array is symmetric. (c) Asymmetric intensity distribution resulting from theLuciusprism array. (d) An image of traced light rays through theLuciusprism array obtained by the simulation tool. (e) Geometry and definition of angles for the refraction through a prism. (f) These two pictures demonstrate a dramatic contrast when theLuciusprism sheet is placed on the screen of an LCD monitor. An example of such a change in transmittance with the viewing angle is shown in Figure 3c, with different values of prism angle α (refer to Fig. 2a ). It is noted that the oblique angle ( θ in ) is 60° in this example because the transmittance is zero, as shown in Figure 2c . A Lucius prism array for the frontal viewing, with a prism angle α of 60°, was fabricated, and the images of Seoul national university (SNU) logo (optical pictures) seen through the Lucius prism are shown from five different viewing angles designated as (i) through (v) in Figure 2d . A video on the transmittance change with the viewing angle is also given in Supplementary Movie 2 . Figure 3: Disproportionation of intensity of incident light. ( a ) A schematic illustration of a Lucius prism sheet placed between a light source and a detector for the disproportionation of incident light intensity. ( b ) Isoluminance contour plot obtained by a simulation tool. Note that the intensity distribution through the normal prism array is symmetric. ( c ) Asymmetric intensity distribution resulting from the Lucius prism array. ( d ) An image of traced light rays through the Lucius prism array obtained by the simulation tool. ( e ) Geometry and definition of angles for the refraction through a prism. ( f ) These two pictures demonstrate a dramatic contrast when the Lucius prism sheet is placed on the screen of an LCD monitor. Full size image Disproportionation of the intensity of incident light Disproportionation of the intensity of incident light can be realized by allowing the prism side of the Lucius prism sheet to face the incident beam, as schematically shown in Figure 3a . Here, a black metal layer of chromium (Cr; 200–300 nm thickness) was obliquely deposited on one side of the prism array. It is clear from the geometry of the prism that the light incident on the left side of the prism array enters the transparent left side, whereas the majority of the light incident on the right side of the prism array is absorbed into the metal layer. This disproportionation of incident light intensity is also clearly demonstrated in the simulation results obtained with LightTools, a simulation package, shown in Figure 3b,c . The result in Figure 3b is for the prism array without a black metal coating, and, as such, the symmetry of light intensity around the apex of the prism is evident. For the Lucius prism shown in Figure 3c , however, the intensity is localized on the left side, with the intensity on the right side being nearly zero. The tracing of the light rays incident perpendicularly to the prism was carried out with LightTools, and the result is shown in Figure 3d . It can be seen that all of the rays from the light source are guided to the left side, whereas a majority of the rays are absorbed on the right side. The direction in which the light intensity is at its maximum can be determined with the aid of Snell's law [1] . Referring to Figure 3e , it follows from this law that where n air and n polymer are the refractive indices of air and polymer, respectively, and the angles α , β and γ are defined in Figure 3e . Note that γ gives the direction in which the intensity is at its maximum. For example, γ is 26° when a typical value of n for polymer, 1.5, is used in equations (4) and (5) for a prism angle α of 45°, with n air =1. Figure 3f shows the brightness contrast resulting from placing the Lucius prism sheet on the screen of a liquid crystal display (LCD) monitor. The left side of the figure shows the view in the direction of the maximum intensity, whereas the right side is in the opposite direction. We note that the bright side has a similar brightness as the background, which serves as a reference for the screen without the sheet, and the dark side is almost non-transparent ( Supplementary Movie 3 ). Autostereoscopic 3D display The ability of the Lucius prism array to directionally allocate the incident light intensity suggests its use in various optical devices [18] , [19] , [20] , [21] , [22] , [23] , [24] , [25] , [26] , such as dual-view or autostereoscopic 3D display [27] , [28] , [29] , [30] , [31] . To perceive a 3D image, human eyes must see different views (binocular disparity), allowing for the sensation of depth known as stereopsis after complicated processing in the brain [29] . Autostereoscopy implies that one can see a different image at each eye without wearing special glasses [27] , [28] , [29] , [30] , [31] . To demonstrate its potential application, we first obliquely deposited a black Cr layer of ~200 nm thickness with a slit-type shadow mask (first metal deposition) on a prism array. Another Cr layer of the same thickness was then deposited in the same way in the opposite direction, while screening the predeposited region by suitably locating the shadow mask (second deposition; Supplementary Fig. S5 ). 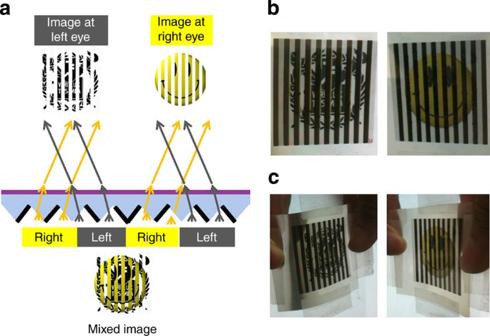Figure 4: Autostereoscopic 3D display. (a) A schematic illustration showing the concept of an autostereoscopic display with theLuciusprism array. When the prism side of theLuciusprism array is placed on a mixed image in good alignment, two distinctively different images are seen by the left and right eyes. (b) Pictures taken from the positions of the left (SNU logo) and right eye (smiley face). (c) Transformation of the printed picture when the flexibleLuciusprism sheet is bent backward (SNU logo) and forward (smiley face) while holding the left-hand side firm. The slit area was 4 cm×4 cm. Subsequently, the Lucius prism array is placed on a picture of two mixed images (smiley face and university logo in this example) with the same slit period as that of the shadow mask slits, as shown in Figure 4a . We mixed the image appearing on the left side of the screen with the image corresponding to the right side with alternating slits containing two different images, one after another. Owing to the disproportionation of light intensity through the slit-type Lucius prism array, one can see only the left image, the university logo in Figure 4a , on the left side, and the right image, the smiley face in Figure 4a , on the right side ( Supplementary Fig. S6 ). Figure 4b shows such separation of the two images when pictures are taken at the positions of left and right eyes ( Supplementary Movie 4 ). The slit size in the present case is large enough that our eyes recognize them in this proof-of-concept demonstration. However, more sophisticated processing equipment than the one employed here can make the size small enough not to be noticed by our naked eyes. With the current optical characteristics, the Lucius prism array can be used for dual-view monitors, showing two different images at both the left and right positions or for small-size autostereoscopic displays typically encountered in mobile phones and handheld game consoles. Figure 4: Autostereoscopic 3D display. ( a ) A schematic illustration showing the concept of an autostereoscopic display with the Lucius prism array. When the prism side of the Lucius prism array is placed on a mixed image in good alignment, two distinctively different images are seen by the left and right eyes. ( b ) Pictures taken from the positions of the left (SNU logo) and right eye (smiley face). ( c ) Transformation of the printed picture when the flexible Lucius prism sheet is bent backward (SNU logo) and forward (smiley face) while holding the left-hand side firm. The slit area was 4 cm×4 cm. Full size image The Lucius prism array possesses several unique features in 3D display when compared with conventional methods. Although autostereoscopy with a prism-patterned screen that is applicable for projection-type display only has recently been reported [32] , the schemes that flat-panel industry currently relies upon for autostereoscopic 3D display [27] , [28] , [29] , [30] , [31] are typically variations of parallax barriers [33] and lenticular lenses [34] for which the origins date back to the 1900s. In the Lucius prism array presented here, the incident light is guided through the prism with directionality so that a different image is viewed at a different position without periodic change of images depending on the viewing angle [31] , which is typically encountered in the two traditional cases ( Supplementary Movie 5 , based on the scheme of parallax barriers). When the images are periodically changed, there are several positions in which human eyes perceive pseudoscopic images (implying the reverse depth perception) or dark regions [31] . In the case of the Lucius prism array, however, such a periodic change of images to the eye does not take place; instead, as schematically drawn in Supplementary Figure S6 , there is a transition from 3D to 2D images at a certain location, without the requirement of time-sequential synchronization of the LCD backlight to the panel demonstrated in other displays [35] . Furthermore, the Lucius prism array would provide an advantage when designing pixels in flat-panel displays because one can make the pixel size with n ( n : integer) times the fixed prism size with a proper change of slit size. We expect that such a modification would be technically less complicated when compared with the fabrication of lens-type structures. The optical directionality of the Lucius prism array can help the user see different images by changing the viewing angle. Figure 4c shows the transformation of a printed picture, a picture of two mixed images, from smiley face to university logo, when the Lucius prism sheet that was bonded to the picture printed on a flexible substrate is bent. When the right-hand side of the sheet is bent backward while holding the left side firm, the SNU logo appears as shown in Figure 4c ( Supplementary Movie 6 ). When the right-hand side is bent in the opposite direction, however, the image is changed to the smiley face. Because the imaging sheet is bendable, the Lucius prism array presented here would be particularly useful for flexible displays [36] , [37] . The Lucius prism array is one in which a part of the prism surface is covered with a reflective or black film. Fully explored here are triangular Lucius prisms, with metal film coverage extended down from the prism apex. Further exploration regarding the prism shape, the prism angles and the metal coverage distribution among prisms could lead to yet uncharted areas. Directional light transmission afforded by the Lucius prism array allows an object to be visible only in the desired direction. By simply placing a Lucius prism sheet on a screen, for example, the screen can be made to permit only frontal viewing, which would be quite useful for security films. The disproportionation of light intensity when rays pass through the Lucius prism array allows the allocation of light in the desired direction. An autostereoscopic 3D display component was demonstrated as a proof-of-principle by fabricating a slit-type Lucius prism array with the help of a shadow mask. Two distinctly different images could be shown to the left and right eyes without the need of special viewing eyewear. Further optimization of the design, such as prism shapes, angles, refractive index, additional optical components and precise alignment control of slit in high resolution, should be addressed to fabricate the Lucius prism array for commercial 3D displays. Fabrication of the prism array The masters used in the present study were prepared mechanically. First, a blank roll or plate of stainless steel electroplated by nickel was prepared. The blank roll or plate surface was machined by a diamond-cutting tool with a specific angle. In this process, the pitch and angle of carved patterns correspond to those of the diamond tool. The height of the patterns depends on the cutting depth of the diamond tool. After the preparation of the masters, drops of a soft PUA (301RM, Minuta Tech) prepolymer solution were dispensed onto the master mould, and a flexible PET film, ~50 μm thick, was placed on top of the mould and lightly pressed against the moulding liquid (PUA) for a supporting backplane. The PUA liquid was then exposed to ultraviolet light for 3 min, with an intensity of 1.7 mW cm −2 . Subsequently, the cured polymer replica was removed from the master. Oblique metal deposition The polymer prism array (50 μm in period, 45° or 60° in prism angle) was coated with 100–300 nm thick Al or Cr metal on one side of the prism using only oblique metal evaporation. We used a thermal and electron gun evaporator for the metal deposition and placed the polymer prism array on an inclined holder with an angle 30–60°. During the deposition, evaporated metal atoms were guided vertically at ~10 −6 Torr, with the inclined holder defining the oblique incidence angle, resulting in the deposition of metal layers only on one side of the prism array. The Lucius prism array thus fabricated had an area of 4×4 cm 2 . To reduce the plasmonic effects from evanescent wave penetration into a metal film, we used Al or Cr as a metal film with a thickness greater than 100 nm [38] . Scanning electron microscopy High-resolution SEM images of the patterns were obtained using Philips XL30FEG. To avoid charging effects, the polymer prism film was sputter coated to 5 nm thickness with Pt before measurement. Simulation of light rays We used a commercial software package (LightTools) for the simulation of optical properties. The simulation was performed for five prism arrays (50 μm in period, 5 mm in length), with a constant refractive index of 1.5 for the polymer. The arrays with different numbers of prisms yielded similar results. We used a Lambertion-type light source in the simulation. Fabrication of the autostereoscopic Lucius prism array We used a slit-type shadow mask to screen a portion of an area. A black metal layer of Cr was first deposited obliquely to a thickness of ~200 nm through the shadow mask. Next, a second layer was deposited in the same way but in the opposite direction, while screening the first-deposited metal layer. The slit area was 4 cm×4 cm. To enhance brightness, the images were printed on a transparent film and bonded to the Lucius prism array on a LCD backlight unit. How to cite this article: Yoon, H. et al . Arrays of Lucius microprisms for directional allocation of light and autostereoscopic three-dimensional displays. Nat. Commun. 2:455 doi: 10.1038/ncomms1456 (2011).